A very stable complex of a modified marine cyclopeptide with chloroform Noncovalent interactions play a pivotal role in molecular recognition. These interactions can be subdivided into hydrogen bonds, cation–π interactions, ion pair interactions and London dispersion forces. The latter are considered to be weak molecular interactions and increase with the size of the interacting moieties. Here we show that even the small chloroform molecule forms a very stable complex with a modified marine cyclopeptide. By means of high-level quantum chemical calculations, the size of the dispersive interactions is calculated; the dispersion energy (approximately −40 kcal mol −1 ) is approximately as high as if the four outer atoms of the guest form four strong hydrogen bonds with the host. This strong binding of chloroform to a modified marine cyclopeptide allows the speculation that the azole-containing cyclopeptides–haloform interaction may play some biological role in marine organisms such as algae. Molecular recognition is a key process in chemistry and biology. Of high interest are noncovalent host–guest interactions that are mainly dominated by London forces [1] , [2] , [3] , [4] , [5] , [6] , [7] . Here an outstanding challenge is the design of host molecules which are able to bind small nonpolar guests, because these types of guests exhibit only weak dispersion interactions owing to their small number of atoms [8] , [9] , [10] . A prominent example for a host system, which includes small nonpolar guests, is the cryptophane family [11] , [12] . Cryptophane cages consist of two C 3 -symmetric cup-shaped cyclotriveratrylene units ( 1 , see Fig. 1 ), which are connected via three mostly aliphatic linkers. Cryptophane-A ( 5 ) is able to bind chloroform with an association constant K i of 230 M −1 at 298 K in C 2 D 2 Cl 4 (refs 13 , 14 ). The by far highest affinity ( K i =3,000 M −1 ) has been measured for the Xe@cryptophane-A complex [15] . It should be noted that the complex formation constants were measured under conditions excluding hydrophobic effects. If these are not excluded, even higher binding constants are found. For example, a water-soluble triacetate-functionalized cryptophane-A derivative shows the highest affinity for xenon, which was ever measured for a host molecule ( K i =33,000 M −1 at 293 K in buffer) [16] . An increase of the association constant can also be obtained by adjusting the cavity to the guest [17] . For example, cryptophane-E ( 6 ) has a slightly larger cavity than cryptophane-A and therefore binds chloroform with a higher association constant ( K i =470 M −1 at 300 K in C 2 D 2 Cl 4 ) [18] , [19] . 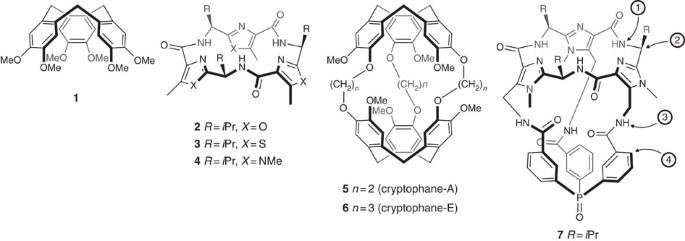Figure 1: Host molecules and their building blocks. Structures of cyclotriveratrylene (1), the azole-containing macrocycles2–4, cryptophane-A (5), cryptophane-E (6) and the imidazole-containing container7. Figure 1: Host molecules and their building blocks. Structures of cyclotriveratrylene ( 1 ), the azole-containing macrocycles 2–4 , cryptophane-A ( 5 ), cryptophane-E ( 6 ) and the imidazole-containing container 7 . Full size image Recently, we dealt with modified marine cyclopeptides (for example, 2 – 4 ), which exhibit three azole units in their cyclopeptidic scaffold and are thus structurally similar to cyclotriveratrylene ( Fig. 1 ) [20] , [21] . The naturally occurring azole cyclopeptides are mainly biosynthesized by cyanobacteria (blue-green algae); the azoles arise from natural amino-acid residues by enzyme-mediated post-translational modification [22] . The in vivo role of these azole-containing cyclopeptides is still unknown, but because of their size and conformation it has been speculated that they are possibly used for metal complexation or as transporting agents [23] . We could show that the spatial structure of the azole-containing macrocycle is strongly dependent on the azole ring [24] . However, in all cases only one conformation exists in solution; this means that an inversion of the macrocycle does not take place. Furthermore, structural investigations of modified marine cyclopeptides revealed that small halogenated hydrocarbons, such as methylene chloride or chloroform, are enclosed into the solid [25] . They are mainly found within the concave cavity, which is formed by the three azole rings. Here we report the properties of the C 3 -symmetric imidazole-containing cyclopeptide cavitand 7 ( Fig. 1 ) as host for chloroform and other 1,1,1-trihalomethanes. One cup-shaped side of container 7 is formed by the imidazole-containing cyclopeptide 4, which is connected via amide bonds to a second cup consisting of a triphenylphosphane oxide unit. NMR investigations reveal that container 7 forms an extremely stable complex with chloroform. High-level quantum chemical calculations show that the dispersive interactions are responsible for the measured complex stability of CHCl 3 @ 7 . Determination of the binding constants The synthesis of 7 was carried out by established protocols [26] in a few steps ( Supplementary Fig. S1 ). For excluding hydrophobic effects and for a better comparison with the already well-known cryptophane compounds 5 and 6 (refs 13 , 18 ), NMR complexing studies of cavitand 7 with chloroform were performed in C 2 D 2 Cl 4 . This solvent is too large to fit within the cavity and guarantees that the receptor 7 is empty. The addition of chloroform to container 7 at 298 K leads to the formation of the inclusion compound CHCl 3 @ 7 and a signal of the enclosed chloroform appears at δ =5.19 p.p.m. in the 1 H NMR spectrum ( Fig. 2a,b ). This highfield shift (Δ δ =2.10 p.p.m.) is consistent with an intramolecular inclusion of the guest into the cavity of 7 . The host signals are also shifted by complexation. If an excess of chloroform is used, the signals of the free host disappear completely ( Fig. 2b ). 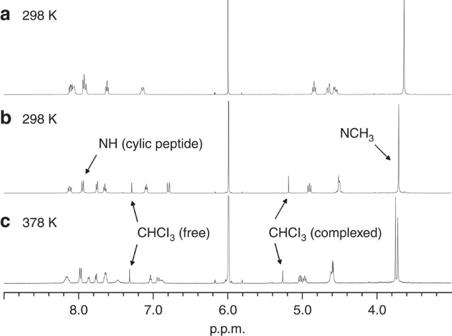Figure 2:1H NMR spectra of 7 and CHCl3@7. The1H NMR spectra of7(a) and CHCl3@7(b,c) were measured at 500 MHz in C2D2Cl4. Figure 2: 1 H NMR spectra of 7 and CHCl 3 @7. The 1 H NMR spectra of 7 ( a ) and CHCl 3 @ 7 ( b , c ) were measured at 500 MHz in C 2 D 2 Cl 4 . Full size image A complete removal of chloroform can only be achieved by heating a diluted solution for several hours in C 2 D 2 Cl 4 at 413 K. As the equilibrium is so strongly shifted to the side of the complex, the thermodynamic parameters were determined by temperature-dependent NMR spectroscopy between 353 and 398 K in C 2 D 2 Cl 4 ( Supplementary Figs S2, S3 and S4 ). At these temperatures and millimolar concentrations, it is guaranteed that a sufficient amount of uncomplexed container 7 is present in solution. The inclusion/exclusion process is, even at these temperatures, so slow that separate 1 H NMR signals for the complex, the host and chloroform are obtained ( Fig. 2c ). For example, integral evaluation at 395 K leads to a binding constant K i of 420 M −1 . The plot of ln K i against 1/ T in the area of 353–398 K furthermore allows the determination of the enthalpy (Δ H i ) and the entropy (Δ S i ) of the inclusion ( Table 1 ). As expected, the inclusion of chloroform by container 7 is strongly enthalpy driven, while the entropy disfavours this process. With the help of enthalpy (Δ H i ) and entropy (Δ S i ), it is also possible to calculate the free enthalpy of inclusion (Δ G i ) and hence the binding constant at 300 K. At this temperature K i amounts to 140,000 M −1 for CHCl 3 @ 7 and is thus more than two orders of magnitude higher than the binding constants for CHCl 3 @ 5 and CHCl 3 @ 6 ( Table 1 ). Table 1 Thermodynamic data determined by 1 H NMR spectroscopy. Full size table To shed light on the role of the solvent in the complex formation, we tried to determine the binding constant in dichloromethane- d 2 , methanol- d 4 and toluene- d 8 . Unfortunately, temperatures equal to or higher than 353 K are needed to reach the equilibrium within a reasonable timescale and the determination of K i could not be performed in pure dichloromethane or methanol. Therefore, dichloromethane (100-fold excess over chloroform) was added to the complex CHCl 3 @ 7 in C 2 D 2 Cl 4 . In this solvent mixture, K i was determined to be 900 M −1 at 353 K ( K i =1,700 M −1 at 353 K in pure C 2 D 2 Cl 4 ). In other words, dichloromethane reduces the binding constant of chloroform by solvent competition, but the effect is not very pronounced. The binding constant in toluene, which, like C 2 D 2 Cl 4, is too large to fit within the cavity, was measured to be 480 M −1 at 359 K ( Table 1 ). The determined enthalpy and the entropy of the inclusion are similar to that found in C 2 D 2 Cl 4 ( Supplementary Fig. S5 ). To test whether the receptor 7 can also include other 1,1,1-trihalomethanes within its cavity, CHCl 2 Br, CHClBr 2 and CHBr 3 were added to a solution of 7 in C 2 D 2 Cl 4 . For CHCl 2 Br and CHClBr 2 , no formation of an inclusion compound was observed at room temperature. The inclusion/exclusion process is so slow that temperatures higher than 383 K are needed to reach equilibrium within a reasonable timescale. The binding constants at 395 K amount to 340 M −1 for CHCl 2 Br and 120 M −1 for CHClBr 2 ( Table 1 ). Thus, the binding constants decrease with increasing size of the guest. The obtained enthalpy (Δ H i ) and the entropy (Δ S i ) of the inclusion for CHCl 2 Br and CHClBr 2 are in the same range as those found for CHCl 3 ( Table 1 and Supplementary Figs S6 and S7 ). For CHBr 3 , no formation of an inclusion compound could be observed even at 410 K, which is likely due to kinetic reasons (too small entrance into the cavity). Conformational analysis of the inclusion complexes The enclosed guest can in principle adopt two orientations, which are as follows: on the one hand, the proton of the trihalomethane can point towards the cup-shaped cyclopeptide; on the other hand, it can point towards the phosphor atom. In the following, the first (second) orientation is labelled with the symbol ↑(↓). The orientation can be determined by two-dimensional (2D) nuclear Overhauser enhancement spectroscopy (NOESY) experiments: The 1 H– 1 H NOESY spectrum of CHCl 3 @ 7 shows a strong cross peak between the proton of the enclosed chloroform and the amide protons (H1) of the azole-containing cyclopeptide ( Fig. 3 ; for numbering see Fig. 1 ), which is an unambiguous proof for the complex ↑CHCl 3 @ 7 . If the distance between the amide proton H1 and the proton of the adjacent methine group H2 is fixed at 2.94 Å, the value of the Cl 3 CH···H1 distance amounts to 2.65 Å. This means that the CHCl 3 proton is not only pointing towards the cup-shaped cyclic peptide but is even located deep within the cone of the peptidic scaffold. The 1 H– 1 H NOESY spectra of CHCl 2 Br@ 7 and CHClBr 2 @ 7 show that here again the proton of the CHX 2 Y molecule point towards the cup-shaped cyclic peptide ( Supplementary Figs S8 and S9 ). Also of interest is the fact that the 1 H NMR signals for the complexes CHCl 2 Br@ 7 and CHClBr 2 @ 7 show C 3 symmetry at 395 K, but not at 298 K ( Supplementary Figs S10 and S11 ). This means that the rotation of the guests is restricted at 298 K because of an energetically favoured position of the guests within the container, which also explains the high loss of entropy by inclusion. 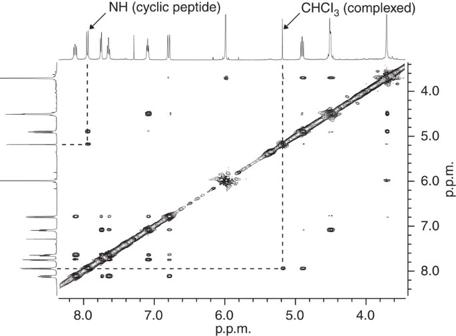Figure 3:Part of the1H–1H NOESY NMR spectrum of CHCl3@7. The NMR spectrum was measured at 500 MHz in C2D2Cl4(298 K). The cross peaks between the proton of the complexed chloroform and the amide protons of the cup-shaped imidazole scaffold are highlighted. Figure 3: Part of the 1 H– 1 H NOESY NMR spectrum of CHCl 3 @7. The NMR spectrum was measured at 500 MHz in C 2 D 2 Cl 4 (298 K). The cross peaks between the proton of the complexed chloroform and the amide protons of the cup-shaped imidazole scaffold are highlighted. Full size image In principle, the triphenylphosphine oxides 7 and CHCl 3 @ 7 can adopt four different conformations ( P1 , P2 , M1 and M2 ): On one side, the three phenyl rings can be present in two opposite helicities ( P or M isomer) and on the other side, the amide protons H3 can point towards ( P1 and M1 ) or away from ( P2 and M2 ) the protons H4 of the phenyl rings (for numbering see Fig. 1 , see also Supplementary Fig. S12 ). To determine the conformations of the free container 7 and the inclusion compound CHCl 3 @ 7 , 2D NOESY and circular dichroism measurements were carried out. For both compounds, cross peaks between the amide protons H3 and the protons H4 of the phenyl rings are found in the 1 H– 1 H NOESY NMR spectra ( Supplementary Figs S13 and S14 ). Furthermore, the circular dichroism spectra of both compounds show negative Cotton effects at 265 nm and positive Cotton effects at 250 nm, which arise from P helicity of the triphenylphosphine oxide chromophore ( Supplementary Fig. S15 ) [26] . These data suggest that the inclusion of chloroform does not lead to a conformational change of the container and both molecules adopt P1 conformation in solution. To support this suggestion, quantum chemical calculations were performed. The structures of all conformers were determined by geometry optimizations at the density functional theory (DFT) level using the MO5-2X functional [27] . The calculations confirm the assumption that only the P1 diastereomers are present in solution ( Supplementary Figs S16 and S17 ). A superimposition of the calculated molecular structures of the empty and the chloroform-filled receptor shows that they are very similar ( Supplementary Fig. S18 ). Calculation of the attractive interaction within CHCl 3 @7 To evaluate the contribution of attractive dispersion forces to the highly negative enthalpy of the inclusion, ab initio calculations were carried out. The molecular structures were optimized using the DFT potential MO5-2X, which has been shown to cover midrange correlation ( Fig. 4 ) [27] . For the light elements C, H, N and O the 6-31G* basis set was used, whereas for the heavy elements P, S and the halogens (F, Cl and Br) the correlation-consistent polarized valence triple-zeta (cc-pVTZ) basis set was employed. On the basis of these geometries, single-point calculations with B3LYP [28] , [29] , [30] and B3LYP-D3 were carried out. While the first method cannot describe the dispersion interaction correctly, especially not at large distances, the latter one includes an additional dispersion correction [31] , [32] , [33] . Thus, the difference between the two is a hint to the extent of the complex dispersion energies. For the light elements C, H, N and O, the 6-311++G** basis set was used, whereas for the heavy elements P, S and the halogens (F, Cl and Br) the aug-cc-pVTZ basis set was employed. The so obtained data are summarized in Table 2 (see also Supplementary Table S1 and Supplementary Data 1 ). 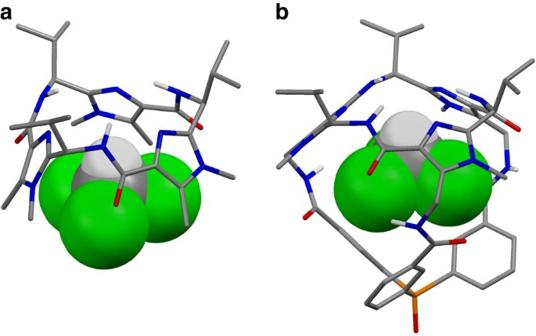Figure 4:Molecular structures of↑CHCl3·4 and↑CHCl3@7. The geometry of the complexes ↑CHCl3·4(a) and ↑CHCl3@7(b) was optimized using MO5-2X/6-31G*,cc-pVTZ. Most hydrogen atoms are omitted for clarity. Figure 4: Molecular structures of ↑ CHCl 3 ·4 and ↑ CHCl 3 @7. The geometry of the complexes ↑CHCl 3 · 4 ( a ) and ↑CHCl 3 @ 7 ( b ) was optimized using MO5-2X/6-31G*,cc-pVTZ. Most hydrogen atoms are omitted for clarity. Full size image Table 2 Calculated interaction energies. Full size table A glance at the table reveals that inclusion of C 2 H 2 Cl 4 by 7 is energetically disfavoured and thus the use of C 2 D 2 Cl 4 as solvent guarantees the exclusion of the solvent from the cavity. As mentioned above, the enclosed chloroform can adopt two orientations. A comparison of the calculated values shows that all methods favour complex ↑CHCl 3 @ 7 . The distance between the proton of the enclosed chloroform and the amide protons of the azole-containing cyclopeptide (H1) is calculated to be 2.886 Å in ↑CHCl 3 @ 7 ; in the energetically disfavoured complex ↓ CHCl 3 @ 7 the distance amounts to 5.712 Å. The first value is consistent with the one found by 1 H– 1 H NOESY NMR measurements (2.65 Å). The binding energies for the complex ↑CHCl 3 @ 7 calculated using MO5-2X and B3LYP-D3 (−20.5 kcal mol −1 and −26.5 kcal mol −1 ) are however significantly higher than the experimentally determined enthalpy of −16 kcal mol −1 . However, it has to be considered that all calculations were carried out for the gas phase, while the experiments were performed in solution (C 2 D 2 Cl 4 ). Assuming that the interactions of the host and the complex with the solvent are similar, only the interaction between chloroform and the solvent molecules has to be taken into account. To simulate this interaction, we calculated the complex formation of two molecules C 2 H 2 Cl 4 and one molecule chloroform (see Table 2 ). If this interaction energy is subtracted from the complex formation energy of ↑CHCl 3 @ 7 , the revised values −15.3 kcal mol −1 (MO5-2X) and −20.2 kcal mol −1 (B3LYP-D3) are obtained, which are now quite similar to the experimentally determined enthalpy of −16 kcal mol −1 . Table 2 shows that the energy values for the complex ↑CHBr 3 @ 7 calculated using MO5-2X and B3LYP-D3 (−19.8 and −29.5 kcal mol −1 ) are similar to those found for the complex ↑CHCl 3 @ 7 . This supports the above-made assumption that the complex formation of CHBr 3 @ 7 at 410 K is prevented by kinetic reasons and not by thermodynamics. According to the calculations, the cyclic peptides 2 – 4 should also form stable complexes with chloroform. Calculated gas-phase interaction energies are approximately from −12 to −13 kcal mol −1 (MO5-2X) and −16 kcal mol −1 (B3LYP-D3). These high values indicate that the cup-shaped imidazoles in 7 are crucial for the formation of the stable complex ↑CHCl 3 @ 7 . Furthermore, for imidazole-containing cyclopeptide 4 , complex energy calculations with CHF 3 and CHBr 3 were carried out. The result is that the interactions are similarly strong and that the orientation of the haloform molecules does not play a major role with the exception of CHF 3 . A comparison of the binding energies for the complex ↑CHCl 3 @ 7 calculated using MO5-2X and B3LYP-D3 (−20.5 and −26.5 kcal mol −1 ) shows that they are significantly higher than those values calculated for the complex formation of chloroform with other arenes. Coupled cluster [CCSD(T)] calculations yield binding energy of −5.46 kcal mol −1 for the chloroform-benzene dimer [34] . A van der Waals density functional study finds a binding energy of −8.22 kcal mol −1 for the adsorption of chloroform on graphene [35] . Attraction in these arene–chloroform complexes mainly derives from the dispersion interaction, whereas the electrostatic contribution is small. A comparison between the interaction energies for ↑CHCl 3 @ 7 calculated with B3LYP and B3LYP-D3 shows that here again the dispersion energy is the crucial term for complex formation. Thus, energy of +7.3 kcal mol −1 is even needed for complex formation of ↑CHCl 3 @ 7 according to B3LYP calculations. Only the consideration of the dispersion correction D3, which amounts to 33.8 kcal mol −1 leads to a stabilization of the complex ↑CHCl 3 @ 7 . The exact extent of dispersion interactions between the monomers in a complex can be obtained via density fitting DFT-symmetry-adapted perturbation theory (DF-DFT-SAPT) calculations [36] , [37] , [38] . However, very large basis sets near saturation (cc-pVQZ, and so on) are necessary for accurate evaluation of the dispersion energy [39] . It is thus not possible to calculate the dispersion energy for the entire system ↑CHCl 3 @ 7 . Therefore, we chose the following two approaches to make a semiquantitative determination of the dispersion energy: for the first approach, we selected a small subsystem, calculated with a very large basis set and extrapolated to the entire system. For the second approach, we chose a large subsystem, which is very similar to ↑CHCl 3 @ 7 , calculated with a medium-size basis set and extrapolated to the result of the very large basis set. As a starting point for the first approach, we chose the MO5-2X-optimized structure of ↑CHCl 3 @ 7 , removed two-thirds of the C 3 -symmetric host as well as the isopropyl group and saturated the unsaturated valencies with hydrogen atoms. The isopropyl group should have no influence on the dispersion energy because it is not a part of the cavity. The obtained model complex CHCl 3 · 8 is depicted in Fig. 5 and should exhibit one-third of the dispersion interactions of system ↑CHCl 3 @ 7 . The DF-DFT-SAPT-calculated dispersion energies for complex CHCl 3 · 8 are listed in Table 3 (see also Supplementary Table S2 ). In all cases, the functional of Perdew, Burke and Ernzerhof (PBE) was used [40] , [41] . As expected, the dispersion energy depends on the used basis set. The largest basis set (aug-cc-pVTZ for C, H, N, O and aug-cc-pVQZ for Cl, P) delivers a value of E Disp =−14.1 kcal mol −1 . After extrapolation to the system ↑CHCl 3 @ 7 the dispersion energy amounts to −42 kcal mol −1 (3 × −14.1 kcal mol −1 ). 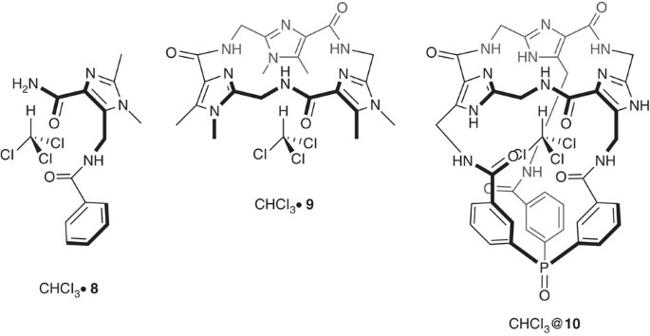Figure 5: Model complexes. The model complexes CHCl3·8, CHCl3·9and CHCl3@10were used for determination of dispersion energy of complex CHCl3@7. Figure 5: Model complexes. The model complexes CHCl 3 · 8 , CHCl 3 · 9 and CHCl 3 @ 10 were used for determination of dispersion energy of complex CHCl 3 @ 7 . Full size image Table 3 Calculated dispersion energies. Full size table Starting point for the second approach of dispersion energy determination in system ↑CHCl 3 @ 7 is also the MO5-2X-optimized structure of ↑CHCl 3 @ 7 . On the basis of this structure, all isopropyl groups as well as three methyl groups were removed, and unsaturated valencies were saturated with hydrogen atoms. The resulting complex CHCl 3 @ 10 ( Fig. 5 ) was calculated with DF-DFT-SAPT. The cc-pVDZ basis set was used for the light elements and the aug-cc-pVQZ basis set for the heavy elements ( Table 3 ). Therefore, an energy value of −33.7 kcal mol −1 is obtained for the dispersion energy. Here it has to be considered that the used basis set does not include the whole dispersion energy. The results for system CHCl 3 · 8 show ( Table 3 ) that only 87% of the dispersion energy calculated with aug-cc-pVTZ,aug-cc-pVQZ are received using the cc-pVDZ,aug-cc-pVQZ basis set. If the dispersion energy of CHCl 3 @ 10 calculated with cc-pVDZ,aug-cc-pVQZ is extrapolated to the larger basis set, the resulting energy value amounts to −39 kcal mol −1 . Both approaches therefore lead to a dispersion energy of about −40 kcal mol −1 in the complex ↑CHCl 3 @ 7 . The results for model complex CHCl 3 · 9 ( Fig. 5 and Table 3 ) furthermore show that the main dispersion energy contribution is caused by the interaction of chloroform and the imidazole-containing macrocycle. The C 3 -symmetric cavitand 7 consisting of a cup-shaped imidazole-containing cyclopeptide, which is connected to a triphenylphosphane unit via amide linkers, was successfully synthesized and characterized. Temperature-dependent NMR investigations showed that this container forms an extremely stable complex with chloroform. The formation constant for this complex is even more than two orders of magnitude higher than the one found for CHCl 3 @cryptophane systems. A reason for the extremely strong complex CHCl 3 @ 7 is the negative enthalpy whose absolute value is twice as high as that for CHCl 3 @ 5 and CHCl 3 @ 6 ( Table 1 ). Ab initio calculations (DFT and DF-DFT-SAPT) revealed that a very high dispersion energy (about −40 kcal mol −1 ) is responsible for the measured complex stability of CHCl 3 @ 7 . As chloroforms has only four interacting atoms (3 × Cl and 1 × H), a dispersion contribution of about −10 kcal mol −1 is found for each outer atom of the guest. It should be mentioned here that strong hydrogen bonds involving neutral species [42] , [43] tend to be in the range of 3–15 kcal mol −1 . Thus, the attractive dispersive interactions between the guest and the host in ↑CHCl 3 @ 7 equal the energy in a scenario where all four outer atoms of the guest form strong hydrogen bonds to the host. An explanation for the high dispersion energy is probably the fact that the trigonal bipyramidal cavity of 7 perfectly fits to the shape of the trihalomethanes. The guests are embedded in such a way that a multitude of dispersion interactions between the trihalomethanes and the atoms of the cavity takes place ( Supplementary Fig. S19 ). The surfaces of the guests and the cavity match in size and shape so perfectly that there is not sufficient space for free rotation of the guests. This is confirmed by the restricted rotation of the guests at 298 K. An analogous effect for cryptophanes showing more spherical cavities has not been observed. A further possible reason for the high stability of CHCl 3 @ 7 compared with that of CHCl 3 @ 5 and CHCl 3 @ 6 may be that the cryptophanes do not completely exclude the solvent and thus the container 7 shows improved size discrimination. The fact that the cup-shaped azole-containing cyclopeptide is mainly responsible for the strong binding of chloroform shows that these cyclopeptides are new recognition units for 1,1,1-trihaloalkanes and prompt speculation that the azole-containing cyclopeptide–haloform interaction might play some biological role. This speculation is supported by the fact that algae and other marine organisms are the largest source of chloroform, bromoform and other biogenic 1,1,1-trihaloalkanes [44] , [45] . General All chemicals were reagent grade and were used as purchased. Reactions were monitored by thin layer chromatography analysis with silica gel 60 F254 thin-layer plates. Flash chromatography was carried out on silica gel 60 (230–400 mesh). 1 H, 13 C NMR and 2D NMR spectra were measured with Bruker Avance DRX 500 and HD 600 spectrometers. All chemical shifts ( δ ) are given in p.p.m. The spectra were referenced to deuterated solvents indicated in brackets in the analytical data. HR-MS spectra were recorded with a Bruker BioTOF III Instrument. The cyclic peptide 11 (ref. 26 ) and the tricarboxylic acid chloride 12 (ref. 46 ), which are starting materials for the synthesis of 7 ( Supplementary Fig. S1 ), were synthesized as reported. Synthesis of 7 To a slurry of cyclic peptide 11 (73 mg, 0.10 mmol) in dry dichloromethane (DCM) (30 mL) a 0.50-M stock solution of 12 in DCM (240 μl, 0.12 mmol) was added at 0–5 °C followed by the slow addition of a 1.00-M stock solution of Et 3 N in dry DCM (1,000 μl, 1.00 mmol). The cooling bath was then removed, and the mixture was stirred for further 16 h at ambient temperature. Solvent was removed in a rotary evaporator in vacuo, and purification of the product was performed by liquid chromatography on silica gel (CH 2 Cl 2 /ethyl acetate/methanol 75/25/0→75/25/15) to yield 18 mg (18%) of 7 as a colourless solid. 1 H NMR (500 MHz, CDCl 3 ): δ 8.15 (ddt, J 1 =11.4 Hz, J 2 =7.9 Hz, J 3 =1.3 Hz, 3 H, -ArH), 7.96 (d, J =8.8 Hz, 3 H, NH), 7.70 (dq, J 1 =7.9 Hz, J 2 =1.3 Hz, 3 H, -ArH), 7.61 (td, J 1 =7.6 Hz, J 2 =2.2 Hz, 3 H, -ArH), 7.04 (dd, J 1 =7.9 Hz, J 2 =4.4 Hz, 3 H, NH), 6.81 (dt, J 1 =13.2 Hz, J 2 =1.3 Hz, 3 H, -ArH), 4.94 (dd, J 1 =10.4, J 2 =8.2 Hz, 3 H, CH), 4.55 (dd, J 1 =14.8 Hz, J 2 =8.2 Hz, 3 H, CH 2 ), 4.49 (dd, J 1 =14.8 Hz, J 2 =4.7 Hz, 3 H, CH 2 ), 3.75 (s, 9 H, NCH 3 ), 2.15–2.08 (m, 3 H, CH), 1.13 (d, J =6.6 Hz, 9 H, CH 3 ), 0.96 (d, J=6.6 Hz, 9 H, CH 3 ); 13 C NMR (125 MHz, CDCl 3 ): δ 169.16, 163.29, 148.37, 135.72 ( J P,C =12.7 Hz), 134.89 ( J P,C =8.0 Hz), 133.30 ( J P,C =12.2 Hz), 133.29, 132.39 ( J P,C =105.9 Hz), 131.05, 130.05 ( J P,C =2.1 Hz), 129.18 ( J P,C =11.2 Hz), 49.7, 34.4, 33.2, 31.0, 19.3, 18.8; 31 P NMR (202.3 MHz, CDCl 3 ): δ 33.2 p.p.m. ; high-resolution mass spectrometry (electrospray ionization-positive) ( m/z ): [M+H] + calcd. for C 51 H 58 N 12 O 7 P, 981.4289; found, 981.4266; [M+Na] + calcd. for C 51 H 57 N 12 NaO 7 P, 1003.4109; found, 1003.4093; [M+CHCl 3 +H] + calcd. for C 52 H 59 Cl 3 N 12 O 7 P, 1099.3433; found, 1099.3504; [M+CHCl 3 +Na] + calcd. for C 52 H 58 Cl 3 N 12 NaO 7 P, 1121.3252; found, 1121.3320. Determination of the thermodynamic parameters To determine the thermodynamic parameters of CHCl 3 @ 7 in C 2 D 2 Cl 4 , cavitand 7 was first dissolved in chloroform and the solvent was then evaporated. The complex CHCl 3 @ 7 was dissolved in tetrachloroethane- d 2 in a concentration of about 1 mM. The NMR samples were heated up to a defined temperature and allowed to equilibrate. According to the 1 H NMR spectra, equilibrium was reached after 2–4 h. The 1 H NMR spectra for determination of the thermodynamic parameters were measured after 6 h and after 1 day. See Supplementary Figs S2, S3 and S4 . To determine the thermodynamic parameters of CHCl 3 @ 7 in toluene- d 8 , cavitand 7 was first dissolved in chloroform and the solvent was then evaporated. The complex CHCl 3 @ 7 was dissolved in toluene- d 8 in a concentration of about 1 mM. The NMR samples were heated up to a defined temperature and allowed to equilibrate over night. See Supplementary Fig. S5 . To determine the thermodynamic parameters of CHCl 2 Br@ 7 (CHClBr 2 @ 7 ), cavitand 7 and CHCl 2 Br (CHClBr 2 ) were dissolved in tetrachloroethane- d 2 in a concentration of about 1 mM. The NMR samples were heated up to a defined temperature and allowed to equilibrate. All measurements were repeated at least twice. See Supplementary Figs S6 and S7 . Computational study All calculations were performed by using the program package Gaussian 09 (ref. 47 ) and MOLPRPO [48] . Geometry optimizations were performed using the DFT potential MO5-2X (ref. 27 ). For the light elements C, H, N and O, the 6-31 G* basis set was used, whereas for the heavy elements P, S and the halogens (F, Cl and Br) the cc-pVTZ basis set was employed. Compounds 2 – 4 and 7 and their corresponding CHX 3 complexes were completely geometrically optimized within the C 3 point group. The inclusion compound C 2 H 2 Cl 4 @ 7 was optimized without any symmetry restriction. On the basis of these geometries, single-point calculations with B3LYP (refs 28 , 29 , 30 ) and B3LYP-D3 were carried out. For the light elements C, H, N and O, the 6-311++G** basis set was used, whereas for the heavy elements P, S and the halogens (F, Cl and Br) the aug-cc-pVTZ basis set was employed. See Supplementary Table S1 and Supplementary Data 1 . Dispersion energies from DF-DFT-SAPT calculations To assess the contribution of the dispersion energy E Disp in the model complexes CHCl 3 · 8 , CHCl 3 · 9 and CHCl 3 @ 10 , we adopted the terminology derived from the SAPT treatment. In this approach, the total interaction energy E SAPT between closed-shell molecules can be obtained as a sum of individual first and second-order interaction terms, namely, electrostatic E (1) elst , induction E (2) ind and dispersion E (2) disp interaction. Each of these terms is accompanied by its exchange counterpart, abbreviated as E (1) exch , E (2) exch-ind and E (2) exch-disp , respectively. The latter terms arise due to electron exchange between the monomers when the molecules are close to each other. Effects of higher than second order in the intermolecular potential can be estimated from the difference δ (Hartee–Fock; HF) of counterpoise-corrected supermolecular HF calculations and electrostatic and induction energies along with their exchange counterparts obtained from static and response HF-level properties. In sum, using the SAPT treatment the total interaction energy E SAPT between closed-shell molecules can be written as: with Thus, the dispersion energy, E Disp , can be calculated as the sum of E (2) disp and E (2) exch-disp . See Supplementary Table S2 . How to cite this article: Haberhauer, G. et al. A very stable complex of a modified marine cyclopeptide with chloroform. Nat. Commun. 4:2945 doi: 10.1038/ncomms3945 (2013).